Deviation from high-entropy configurations in the atomic distributions of a multi-principal-element alloy The alloy-design strategy of combining multiple elements in near-equimolar ratios has shown great potential for producing exceptional engineering materials, often known as ‘high-entropy alloys’. Understanding the elemental distribution, and, thus, the evolution of the configurational entropy during solidification, is undertaken in the present study using the Al 1.3 CoCrCuFeNi model alloy. Here we show that, even when the material undergoes elemental segregation, precipitation, chemical ordering and spinodal decomposition, a significant amount of disorder remains, due to the distributions of multiple elements in the major phases. The results suggest that the high-entropy alloy-design strategy may be applied to a wide range of complex materials, and should not be limited to the goal of creating single-phase solid solutions. Intermetallic compounds—ordered structures of two or more metallic elements—have long been studied and developed for high-temperature applications [1] , [2] , [3] , [4] . More recently, the high-entropy alloy-design strategy has emerged [5] , [6] , [7] , [8] , in which five or more elements are mixed in near-equimolar ratios, such that the high configurational entropy of mixing could promote solution formation. At high temperatures, disordered solid solutions are especially favoured in such alloys because of the high mixing entropy effect. As temperature decreases, the high-entropy effect becomes less important in relation to the enthalpy effect, and phases with a higher degree of order are favoured, including ordered solid solutions [9] . However, there is still an enhancement of the overall disorder due to the entropy effect, as reflected in the multi-element composition in most phases. Depending on the detailed entropy–enthalpy balance, a number of phases may evolve as the alloy cools from high temperatures, including a random solid solution, partially ordered solid solution, ordered solid solution or even a stoichiometric compound. The present work examines the structural evolution of the Al 1.3 CoCrCuFeNi alloy, from the liquid to the room temperature phases, using integrated experimental to theoretical techniques. The observed phases, including the disordered and partially ordered solid solution structures, are quantitatively described within a unified structural model. This approach goes beyond the common practice of discretely categorizing the phases as ordered versus disordered structures and may lead to a better understanding of the temperature-dependent structures in a wide variety of complex alloys. The term ‘high-entropy’ has been used for alloys with multiple principal elements (that is, five or more elements, with concentrations between 5 and 35 atomic percents) because of their inherent high configurational entropy of mixing in the random solution state and because of the emphasis on enhancing the formation of solid solution phases [5] , [6] . However, to avoid the possible confusion in the discussion of entropy and enthalpy effects on phase separation, or the degree of ordering, the phrase, ‘multi-principal-element alloy’, will be substituted for high-entropy alloy in the discussion below. Many multi-principal-element alloys have shown exceptional properties, including high strengths at elevated temperatures [6] , [8] , [10] , [11] , [12] , [13] , [14] , [15] , ductility [16] , [17] , toughness [18] , resistance to corrosion [19] , [20] , wear [21] and fatigue [22] . These favourable properties are sometimes associated with the locally strained solid solution structures, especially those with simple, single-phase microstructures [5] , [23] , [24] . Given the importance of these structures, and the frequent deviations from them, there is a need to rigorously characterize the atomic distributions, going beyond a basic ‘ordered’ versus ‘disordered’ categorization, to understand the temperature-dependent ordering behaviour. This understanding may be achieved by combining advanced techniques, such as in situ neutron scattering, high-energy synchrotron X-ray diffraction, atom-probe tomography (APT), high-resolution electron microscopy and ab initio molecular dynamics (AIMD) simulations. A randomly mixed solid solution will have a high configurational entropy of mixing , given for ideal solutions by [25] Here, R is the ideal gas constant and x i is the molar fraction concentration of the i th element. For equimolar alloys, this equation reduces to , where n is the number of elements. This simple relationship between the configurational entropy of mixing and the number of principal elements serves as the basis for defining high-entropy alloys as having five or more multiple principal elements [6] . Although the random mixing of n ≥5 elements would result in large values of , the presence of all of these elements does not always ensure that such mixing is achievable or thermodynamically stable [26] , [27] . Phase stability depends on both the entropy and enthalpy, according to the Gibbs free energy, Δ G , which has the general form, where the Δ H is the total enthalpy change, relative to a standard state, and the Δ S is the total entropy change, including both configurational and dynamical contributions [28] . The stable phase always has the lowest Δ G , but not necessarily the largest Δ S (or ). However, is an essential consideration in the design of alloys with multiple principal elements and it is the main focus of the present work. For binary intermetallic compounds, the quantity may be expressed as a function of a site-ordering parameter, η , which ranges from 0 to 1. This model includes the random ( η =0) and fully ordered ( η =1) configurations as limiting cases [1] , [29] , [30] . Here this approach is extended to the case of a multi-principal-element phase by applying a set of order parameters, η i , for i =1 to n elements, which are distributed on two equivalent sublattices (see Methods). The order parameters will now range from −1 to 1, and Equation (1) may then be rewritten, as In the case of a multiphase material, such as the present alloy, the total may be found by the weighted sum of each phase, particularly if no significant volume change occurs due to the phase separation [25] . In the present study, the Al 1.3 CoCrCuFeNi alloy is shown to deviate from the random mixing behaviour, even in the liquid state, according to both simulations and experiments. The solid alloy contains partially ordered phases, where , using equation (3) with the experimental values of η i , measured over a wide temperature range. Although the values are diminished from that of a random solid solution, their finite values demonstrate that the high-entropy alloy-design strategy has significantly influenced the formation of the ordered phases. We conclude that the high-entropy alloy-design strategy should be considered for a broad range of alloy-development problems, far beyond the recent emphasis on single-phase solid solutions. Room temperature microstructures On the scale of hundreds of microns, the microstructure appears as large (~200 μm) crystal grains, representing 95% of the volume fraction, with irregular-shaped islands dispersed throughout the matrix, representing the remaining 5% of the volume ( Fig. 1a ). Although dendritic growth is not obvious from the present microstructure, it is known to occur in the Al x CoCrCuFeNi system, over a wide range of aluminium contents, x (ref. 31 ). Here it is inferred that the dendrites have grown and merged, during cooling from the melt, to form the large-grain microstructure. The irregular-shaped islands represent the remnants of the interdendritic regions. 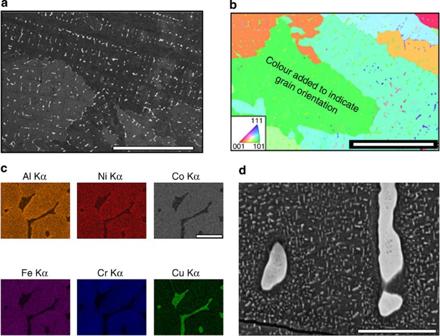Figure 1: SEM. (a) The Al1.3CoCrCuFeNi alloy has large crystal grains (hundreds of microns), with irregular-shaped islands dispersed throughout and between the grains, which is visible at low magnification. The small islands are Cu-rich FCC phases and are actually the interdendritic regions formed during the dendritic crystal growth. Scale bar, 200 μm. (b) A SEM–EBSD map of Al1.3CoCrCuFeNi is colour coded according to the crystal-grain orientations. The matrix is composed of large BCC/B2 grains, and the small islands are FCC structures. Scale bar, 200 μm. (c) An EBSD map highlights the contrast between the BCC/B2 grains and the FCC interdendritic regions in terms of elemental concentrations. The BCC/B2 grains have significant amounts of all the elements (Al, Co, Cr, Fe and Ni), except Cu, which has segregated into the interdendritic regions. Scale bar, 20 μm. (d) X-ray EDS showing that the large crystal grains contain significant amounts of all elements, except Cu, which strongly segregates to the interdendritic regions. Scale bar, 10 μm. Figure 1: SEM. ( a ) The Al 1.3 CoCrCuFeNi alloy has large crystal grains (hundreds of microns), with irregular-shaped islands dispersed throughout and between the grains, which is visible at low magnification. The small islands are Cu-rich FCC phases and are actually the interdendritic regions formed during the dendritic crystal growth. Scale bar, 200 μm. ( b ) A SEM–EBSD map of Al 1.3 CoCrCuFeNi is colour coded according to the crystal-grain orientations. The matrix is composed of large BCC/B2 grains, and the small islands are FCC structures. Scale bar, 200 μm. ( c ) An EBSD map highlights the contrast between the BCC/B2 grains and the FCC interdendritic regions in terms of elemental concentrations. The BCC/B2 grains have significant amounts of all the elements (Al, Co, Cr, Fe and Ni), except Cu, which has segregated into the interdendritic regions. Scale bar, 20 μm. ( d ) X-ray EDS showing that the large crystal grains contain significant amounts of all elements, except Cu, which strongly segregates to the interdendritic regions. Scale bar, 10 μm. Full size image Several grains were individually analysed using a scanning electron microscope, electron-backscatter diffraction (SEM–EBSD) method. The cubic structures and the orientations of individual grains were measured, as shown by the colour coding in Fig. 1b . The crystal structure of these large grains is basically body-centred cubic (BCC), although further details are found on closer examinations, as discussed below. The interdendritic regions have the face-centred cubic (FCC) structure ( Supplementary Fig. 1 ). On the tens-of-microns scale, the X-ray energy-dispersive spectrometry (EDS) reveals that the crystal grains contain an inhomogeneous mixture of all the constituent elements and that interdendritic regions are Cu rich ( Fig. 1c ). The inhomogeneity of the crystal grains is partly due to the presence of hundreds of Cu-rich precipitates, which are distinct from the interdendritic regions ( Fig. 1d ). The combined area fraction of these Cu-rich features (interdendritic regions and rod-shaped precipitates) in Fig. 1d is 15%. The corresponding volume fractions of the interdendritic regions and rods, found by analysing multiple images ( Supplementary Fig. 2 ), are 5 and 10%, respectively. On the submicron level, the microstructure is determined using the high-resolution SEM ( Fig. 2a ), transmission electron microscopy (TEM) and selected area diffraction ( Supplementary Fig. 3 ). The large crystal grains are actually composed of coherent BCC/B2 phase mixtures, where B2 is an ordered variant of the BCC structure, often associated with intermetallics [30] , [32] . The rod-shaped FCC precipitates are dispersed in BCC/B2 grains ( Figs 1d and 2a ). The X-ray EDS shows that Al and Ni are found almost exclusively in the B2 regions, Cr in the BCC regions and Cu in the FCC regions (interdendritic regions and rod-shaped precipitates). Co and Fe, however, are found in both the B2 and BCC regions ( Fig. 2b ). Thus, the room temperature B2 phase contains four principal elements (that is, having concentrations >5 atomic percents) [6] of Al, Ni, Co and Fe. The BCC phase has three principal elements (Cr, Co and Fe), and the FCC phases mainly contain Cu. 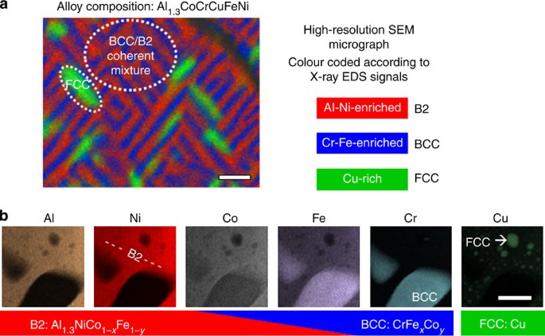Figure 2: Microscopy and elemental analyses. (a) The high-resolution SEM micrograph is colour coded according to EDS, highlighting how the elements segregate and enrich the room temperature phases (B2, BCC and FCC). Scale bar, 0.5 μm. (b) The abundance of each individual element is shown in a series of TEM/EDS images of the same sample region. The selected sample area includes a contiguous B2 region, with two rectangular (roughly) BCC phases, at the bottom and left side, and smaller circular FCC nanopreciptitates. The EDS reveals that Al and Ni are nearly exclusive to the B2 phase (that is, the other regions appear black), Co and Fe are present in both the B2 and BCC phases and Cr is nearly exclusive to the BCC phase. Cu is found nearly exclusively in the nanopreciptitates, which are FCC or ordered variants. The larger FCC interdendritic regions and rod-shaped precipitates, not shown here, also contain mostly Cu. Scale bar, 0.1 μm. Figure 2: Microscopy and elemental analyses. ( a ) The high-resolution SEM micrograph is colour coded according to EDS, highlighting how the elements segregate and enrich the room temperature phases (B2, BCC and FCC). Scale bar, 0.5 μm. ( b ) The abundance of each individual element is shown in a series of TEM/EDS images of the same sample region. The selected sample area includes a contiguous B2 region, with two rectangular (roughly) BCC phases, at the bottom and left side, and smaller circular FCC nanopreciptitates. The EDS reveals that Al and Ni are nearly exclusive to the B2 phase (that is, the other regions appear black), Co and Fe are present in both the B2 and BCC phases and Cr is nearly exclusive to the BCC phase. Cu is found nearly exclusively in the nanopreciptitates, which are FCC or ordered variants. The larger FCC interdendritic regions and rod-shaped precipitates, not shown here, also contain mostly Cu. Scale bar, 0.1 μm. Full size image The BCC/B2 phase mixture is formed by periodic composition modulations within the coherent crystal grains, which is a characteristic feature of spinodal decomposition [25] . The resulting plate-like microstructure has a ~0.2 μm periodicity ( Fig. 2a ) and a significantly-reduced configuration entropy of mixing, compared with a homogeneous BCC phase. Note that similar modulated microstructures have previously been identified in the Al x CoCrCuFeNi alloys and are attributed to spinodal decomposition [31] . These features occur in the high aluminium content compositions (0.8< x <3.0) below the spinodal decomposition temperatures near 600 °C. The Cu segregation occurs on different length scales. The largest Cu-rich structures are the interdendritic regions ( Fig. 1c ), comparable to those previously reported in the Al x CoCrCuFeNi system, which contain between 60 and 80 atomic percent Cu [33] . The interdendritic regions form directly from the Cu-rich liquid, which coexists with the primary BCC phase. The present SEM–EBSD analyses indicate that the interdendritic regions are FCC structures ( Supplementary Fig. 1 ), and EDS shows that they are Cu rich ( Fig. 1c,d ). Two types of submicron Cu-rich precipitates are identified, particularly the rod-shaped ( Fig. 2a ) and spherical nanoprecipitates ( Fig. 2b ). The rods are dispersed throughout the dendrites (that is, the BCC/B2 matrix), but the spheres are found only in the spinodal B2 phase. Given that the total volume of Cu in the material is 16%, it may be inferred that the volume fraction of the Cu nanoprecipitates is on the order of 1% (from above, the Cu-rich rods and interdendritic regions account for 15%). Taking all of the above Cu-rich FCC phases into account, the adjusted volume phase fractions of the alloy are 50% B2, 34% BCC and 16% FCC structures. Despite the distinct types of Cu-rich precipitates observed, the neutron diffraction patterns contain only a single family of FCC peaks (in addition to the B2/BCC peaks), with a room temperature lattice parameter a =3.624±0.003 Å. This structure is similar to the pure Cu (ref. 34 ), which is FCC, with a =3.615 Å. Furthermore, the intensities of the FCC neutron diffraction peaks are consistent with an FCC phase fraction formed by all (or most) of the Cu in the alloy. Because of the above observations, the Cu-rich regions (large and small) are approximated as the pure Cu, having . Several types of Cu-rich precipitates have been reported in the Al x CoCrCuFeNi system, including the FCC, BCC, L1 2 and B2 structures [31] , [33] . Thus, the present approximation may overlook many details of the Cu-segregation behaviour, which is obviously quite complex. Regardless of the details, however, it may be inferred that the Cu segregates in stages during cooling and serves as an important indicator of the overall temperature dependence of . APT provides further details of the elemental distributions, allowing individual atoms to be resolved and colour coded according to the elemental type ( Fig. 3a ). Features, such as the elemental partitioning of the room temperature B2 phase and the appearance of Cu-rich precipitates, much smaller than those described above, are shown in a proximity histogram constructed across the B2–FCC interface ( Fig. 3b ). The Cr-rich precipitates are visible in the atom map ( Fig. 3a ), consistent with other studies [33] . In general, the APT studies verify the multi-component nature of the major phases and detect both copper and chromium nanoprecipitates. These detailed results reveal a seemingly complex microstructure, particularly at room temperature. However, the main trends (composition modulations and elemental precipitations within a solid solution) are quite simple. 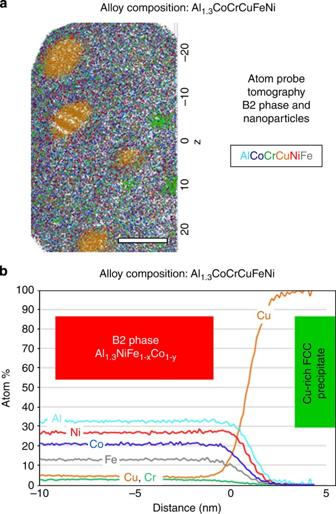Figure 3: APT. (a) An atom map shows the atomic distribution within the B2 phase, which contains Cu-rich and Cr-rich nanoprecipitates. Scale bar, 0.01 μm. (b) Proximity histogram presenting atomic concentrations across the B2–FCC interface. Figure 3: APT. ( a ) An atom map shows the atomic distribution within the B2 phase, which contains Cu-rich and Cr-rich nanoprecipitates. Scale bar, 0.01 μm. ( b ) Proximity histogram presenting atomic concentrations across the B2–FCC interface. Full size image The above results establish the important details of the room temperature microstructure and the phase compositions ( Table 1 ). The crucial information about the site ordering, and the structural evolution with respect to temperature, is obtained through the additional experimental and theoretical analyses, described below. Table 1 Phase compositions. Full size table Complementary neutron and X-ray scattering studies We were unable to directly solve the atomic distributions by performing diffraction experiments and applying Rietveld refinements [35] . There are too many fitting parameters, without a strong refinement convergence. However, here we show that the problem may be reduced to that of refining a single ‘contrast’ parameter (see Methods), which is directly related to the intensity ratio of the superstructure and fundamental reflections. These intensity ratios are generally different for X-rays versus neutrons. Thus, the two experimental techniques provide complementary information. Ultimately, the actual elemental distributions may be inferred from the integrated analyses of the contrast parameters and the microscopy results, described above. Several neutron and synchrotron X-ray diffraction scans were collected in the temperature range of 20 to 800 °C, which are of great interest, because the spinodal transformation possibly occurs [31] near 600 °C. The spinodal microstructure produces overlapping BCC and B2 Bragg reflections, particularly those marked by the solid squares in Fig. 4a , which are common to both the BCC and B2 structures (that is, the fundamental peaks). Peaks marked by the open squares are exclusive to the B2 structure (that is, the superstructure peaks). The Cu-rich interdendritic regions and rods produce the FCC peaks, marked by the solid triangles, which coexist with the BCC/B2 peaks throughout the present temperature range ( Fig. 4a–c ). 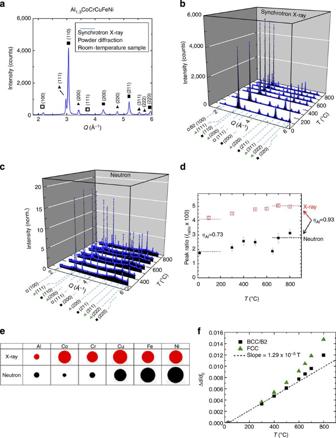Figure 4: Complementary synchrotron X-ray and neutron diffraction results from room temperature to 800 °C. (a) Synchrotron X-ray powder diffraction pattern at room temperature showing the fundamental BCC reflections (solid squares), superstructure BCC_B2 reflections (open squares) and FCC reflections (triangles). (b) A series of synchrotron X-ray powder patterns from 100 to 800 °C. All of the peaks persist throughout the temperature range, without any large changes in the integrated intensities or peak positions. The noticeable increase in the peak heights, with increasing temperature, is accompanied by a decrease in the width and is attributed to the strain relaxation in the fine powder sample. (c) A series of neutron powder patterns from 300 to 800 °C for a solid, polycrystalline sample with sharp peaks (no strain broadening). As found in the X-ray study, all of the peaks persist without any large changes in the integrated peak intensities or peak positions. (d) Integrated intensity ratios of the BCC/B2 (1 0 0) superstructure and (1 1 0) fundamental reflections,Iratio, are plotted versus temperature, for both the synchrotron X-ray and neutron diffraction results. The values are determined from the least-squares fitting of Gaussian curves to the observed peaks, and the error bars from the s.e. of the Gaussian fits. The fitted values are compared with the model calculations, indicated by the dashed black (neutron calculations) and red (X-ray calculations) lines. (e) A schematic comparison of the X-ray and neutron scattering strengths of the elements is shown to demonstrate why the neutron and X-ray peak ratios are so different. (f) The thermal expansion trend, expressed in terms of the change ind-spacing (Δd) divided by the room temperatured-spacing (d0), of the BCC/B2 phases (black squares) is nearly linear (dashed line) below 600 °C. Although the thermal expansion rates increase above 600 °C, no discrete jumps are seen in either the BCC/B2 or the FCC (green triangles) phases. Figure 4: Complementary synchrotron X-ray and neutron diffraction results from room temperature to 800 °C. ( a ) Synchrotron X-ray powder diffraction pattern at room temperature showing the fundamental BCC reflections (solid squares), superstructure BCC_B2 reflections (open squares) and FCC reflections (triangles). ( b ) A series of synchrotron X-ray powder patterns from 100 to 800 °C. All of the peaks persist throughout the temperature range, without any large changes in the integrated intensities or peak positions. The noticeable increase in the peak heights, with increasing temperature, is accompanied by a decrease in the width and is attributed to the strain relaxation in the fine powder sample. ( c ) A series of neutron powder patterns from 300 to 800 °C for a solid, polycrystalline sample with sharp peaks (no strain broadening). As found in the X-ray study, all of the peaks persist without any large changes in the integrated peak intensities or peak positions. ( d ) Integrated intensity ratios of the BCC/B2 (1 0 0) superstructure and (1 1 0) fundamental reflections, I ratio , are plotted versus temperature, for both the synchrotron X-ray and neutron diffraction results. The values are determined from the least-squares fitting of Gaussian curves to the observed peaks, and the error bars from the s.e. of the Gaussian fits. The fitted values are compared with the model calculations, indicated by the dashed black (neutron calculations) and red (X-ray calculations) lines. ( e ) A schematic comparison of the X-ray and neutron scattering strengths of the elements is shown to demonstrate why the neutron and X-ray peak ratios are so different. ( f ) The thermal expansion trend, expressed in terms of the change in d -spacing (Δ d ) divided by the room temperature d -spacing ( d 0 ), of the BCC/B2 phases (black squares) is nearly linear (dashed line) below 600 °C. Although the thermal expansion rates increase above 600 °C, no discrete jumps are seen in either the BCC/B2 or the FCC (green triangles) phases. Full size image As the alloy is heated to 800 °C, the main features of the diffraction patterns persist, including the synchrotron X-ray ( Fig. 4b ) and neutron ( Fig. 4c ) superstructure reflections. The ratios of the BCC/B2 (1 0 0) superstructure and the BCC/B2 (1 1 0) fundamental integrated peak intensities ( I ratio ) were examined using both synchrotron X-ray and neutron diffraction ( Fig. 4d ). The difference between the X-ray and the neutron I ratio values arises from their different scattering behaviours ( Fig. 4e ). Several atomic distribution models were constructed and compared against the observed I ratio values. The best match to the room temperature data is a distribution in which the Al atoms preferentially occupy the α sublattice ( η Al =0.73), the Fe atoms weakly prefer the α sublattice ( η Fe =0.24) and the Ni and Co atoms preferentially occupy the β sublattice ( η Co,Ni =−0.60). No significant amounts of Cr or Cu are present in the spinodal B2 phase. The present order parameters satisfy the constraint that both sublattices have an equal number of atoms (equation 13) and give a good empirical fit to the observed data. The I ratio values ( Fig. 4d ) increase with temperature, except for the dip around 600 °C, which is most pronounced in the neutron data. The I ratio trend indicates a gradual strengthening of the B2 order, and decrease in the , as the spinodal microstructure is heated. This entropy decrease is thermodynamically favourable only if it produces an offsetting benefit, such as lattice-strain minimization, as may be expected in multi-element spinodal alloys [36] . The overlapping B2 and BCC peaks in the present diffraction data indicate that close lattice–parameter matching is indeed maintained in the spinodal microstructure, even as the lattice parameters change with temperature ( Fig. 4f ). The BCC/B2 phases undergo a smaller thermal expansion than the Cu-rich FCC phases, based on the diffraction peak positions and associated d -spacings. The dashed line ( Fig. 4f ) represents a linear fit to the BCC/B2 results, from room temperature to 600 °C. Although the slope increases above 600 °C, no discontinuity in the d -spacing trend is observed. This finding is consistent with the expected spinodal transformation, which occurs by a continuous redistribution of elements on the cubic lattice [37] . Significant changes in the atomic distributions are expected in the temperature range where the I ratio dip is observed ( Fig. 4d ), in the neighbourhood of 600 °C, corresponding to a transition from the spinodal BCC/B2 microstructure to a high-temperature B2 matrix. The dip is much more pronounced in the neutron data, indicating that the transition-metal (TM) elements undergo a significant redistribution. Despite the increased mixing at temperatures above 600 °C, inhomogeneity may persist in the high-temperature ‹B2› matrix, possibly in the form of BCC and B2 domains, as found in the room temperature AlCoCrCuFeNi alloys solidified by rapid quenching [33] . Thus, the notation ‹B2› is used to emphasize that the space-averaged B2 structure is being reported here. In particular, the ‹B2›-order parameters are η Al =0.93 and η TM =−0.29. The negative value of η TM indicates that the TM elements preferentially occupy the β sublattice. The resulting ‹B2› configurational entropy of mixing, , is considerably greater than that of the spinodal microstructure, where . High-temperature neutron scattering studies Neutron scattering on Al 1.3 CoCrCuFeNi was conducted from ambient temperature to 1,400 °C ( Fig. 5a ), a liquid state, using aerodynamic levitation and laser heating ( Supplementary Fig. 4 ) [38] , [39] . The B2 superstructure reflection persists all the way to 1,150 °C ( Fig. 5b ). At higher temperatures, the diffraction intensities (superstructure and fundamental reflections) are too weak to analyze the long-range structure. The primary phase is, therefore, identified as a disordered BCC solid solution. However, the solid solution may have local B2 ordering, similar to the AIMD-simulated results for the liquid phase, discussed below. 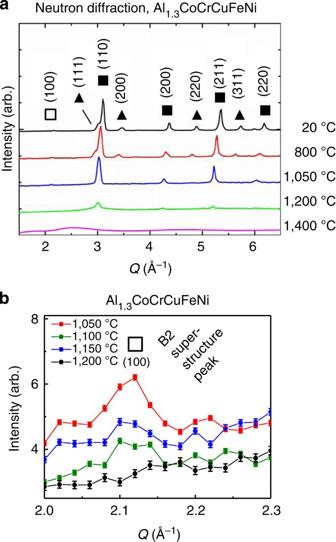Figure 5: Neutron diffraction from room temperature to a molten state. (a) Data were fit to the BCC/B2 and FCC structures, and the corresponding peaks are denoted by squares and triangles, respectively. The open square is used for the ‘superstructure’ reflection, which is extinct in the disordered BCC phase, and the solid squares for the fundamental reflections common to both the BCC and B2 structures. (b) The weak B2 (1 0 0) superstructure peak is present at temperatures at least up to 1,150 °C. The error bars are calculated based on the number of observed neutron counts. Figure 5: Neutron diffraction from room temperature to a molten state. ( a ) Data were fit to the BCC/B2 and FCC structures, and the corresponding peaks are denoted by squares and triangles, respectively. The open square is used for the ‘superstructure’ reflection, which is extinct in the disordered BCC phase, and the solid squares for the fundamental reflections common to both the BCC and B2 structures. ( b ) The weak B2 (1 0 0) superstructure peak is present at temperatures at least up to 1,150 °C. The error bars are calculated based on the number of observed neutron counts. Full size image To understand the local-ordering behaviour, pair distribution function (PDF) analyses of the neutron diffraction data were carried out [40] , [41] , [42] . At room temperature ( Fig. 6a ), the observed PDF approximately matches the periodic atomic arrangement associated with the present cubic crystal structures (B2, BCC and FCC). Here, the fitting model, implemented using the PDFgui software package [43] , represents the ideal structure, where the equilibrium position of each atom falls exactly on its assigned lattice site. Comparing with the observed PDF, the greatest mismatch occurs at short distances, less than 10 Å, suggesting the presence of local lattice distortions due to different atomic sizes in the solid solution [24] . Over long distances, the cumulative effect of the local static distortions is similar to that of thermal displacements, which do not destroy the periodicity of the crystal structure. Thus, the observed PDF matches well with the ideal model (which includes random, thermal displacements) at large distances ( Fig. 6a ). 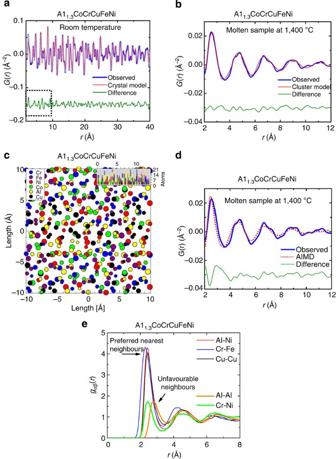Figure 6: The local structure of Al1.3CoCrCuFeNi. (a) The room temperature neutron PDF data (blue), and the calculated43PDF results (red), based on the expected cubic crystal structure, that is, the atomic distances, defined by the unit cell and long-range lattice periodicity, agree reasonably well at large distances,r. As shown by the difference curve (green), and highlighted by the dashed rectangle, the agreement below 10 Å is less than that at larger distances. This trend is consistent with the expectation that HEAs are locally strained24and yet possess long-range crystal order. (b) At 1,400 °C, the observed PDF (blue) shows short-range order, consistent with a liquid phase, and agrees roughly with a model (red) based on local structures (<20 Å diameters) composed of B2 and FCC cells. (c) A snapshot of the liquid structure, at 1,400 °C, was created using AIMD simulations. (d) The observed (blue) and AIMD-simulated (red) PDFs show reasonable agreement at 1,400 °C. (e) Selected partial pair correlation functions,gαβ(r), simulated using AIMD, indicate that some pairs (for example, Al-Ni, Cr-Fe and Cu-Cu) are much more likely to be found as nearest neighbours than others (for example, Al-Al and Cr-Ni). Such preferred nearest-neighbour pairing in the liquid phase is consistent with the formation of a B2-ordered solid solution primary phase, which is supported by the presence of superstructure peaks in the high-temperature diffraction data (Fig. 5a,b). Figure 6: The local structure of Al 1.3 CoCrCuFeNi. ( a ) The room temperature neutron PDF data (blue), and the calculated [43] PDF results (red), based on the expected cubic crystal structure, that is, the atomic distances, defined by the unit cell and long-range lattice periodicity, agree reasonably well at large distances, r . As shown by the difference curve (green), and highlighted by the dashed rectangle, the agreement below 10 Å is less than that at larger distances. This trend is consistent with the expectation that HEAs are locally strained [24] and yet possess long-range crystal order. ( b ) At 1,400 °C, the observed PDF (blue) shows short-range order, consistent with a liquid phase, and agrees roughly with a model (red) based on local structures (<20 Å diameters) composed of B2 and FCC cells. ( c ) A snapshot of the liquid structure, at 1,400 °C, was created using AIMD simulations. ( d ) The observed (blue) and AIMD-simulated (red) PDFs show reasonable agreement at 1,400 °C. ( e ) Selected partial pair correlation functions, g αβ ( r ), simulated using AIMD, indicate that some pairs (for example, Al-Ni, Cr-Fe and Cu-Cu) are much more likely to be found as nearest neighbours than others (for example, Al-Al and Cr-Ni). Such preferred nearest-neighbour pairing in the liquid phase is consistent with the formation of a B2-ordered solid solution primary phase, which is supported by the presence of superstructure peaks in the high-temperature diffraction data ( Fig. 5a,b ). Full size image At the highest temperature studied, 1,400 °C, the observed PDF peaks diminish at distances beyond r ~15 Å, consistent with a liquid phase ( Fig. 6b ). The observed profile at 1,400 °C shows reasonably good agreement with a model having short- and medium-range order, as recently found in ternary liquid metals containing aluminium [44] . The local structure of the liquid is similar to that of the solid, which is modelled using a mixture of BCC and FCC unit cell clusters. It is significant to note that the BCC or FCC cell clusters, alone, do not provide a good fit. Only in combination do they provide a reasonable fit, consistent with recent studies of binary liquid alloys containing mixed cluster types [45] . Interestingly, the mixed clusters in the liquid may be viewed as precursors to the phase segregation in the solid. The mixed cluster model was implemented in PDFgui using the spherical shape factor option. The cluster diameter was used as a fitting parameter, producing the best fits in the range of 5–20 Å. The BCC and FCC cells are randomly populated by all six elements in the alloy, with lattice parameters of 3.00 and 3.801 Å, respectively. The BCC volume phase fraction of 62% and FCC fraction of 38% yield a calculated density of 6.28 g cm −3 . The present PDF experiments show an interesting connection between the short- and medium-range structures of the liquid and solid phases. Many questions remain, however, about the details of the structural and chemical order. For example, the experimentally observed peak splitting in the liquid is not yet well matched by the models. This challenging problem will likely be the subject of many future studies. AIMD simulations The AIMD simulations can predict the local atomic structure of the liquid and give insight into the solidification behaviour of complex alloys [46] , [47] . In the present study, AIMD simulations were run, both with and without constraints from the experimental input. An AIMD ‘snapshot’ of the liquid structure at 1,400 °C is shown in Fig. 6c . The simulated PDF gives a reasonable match with the observed one ( Fig. 6d ), when constrained to match the density (6.28 g cm −3 ) obtained from the experimental fit ( Fig. 6b ). The unconstrained AIMD predicts a higher density, with peaks shifted to smaller pair separations, r . Both the constrained and unconstrained AIMDs, however, predict the same chemical short-range order (CSRO) trends, described below. The AIMD-simulated PDF may be separated into the partial pair correlation functions ( g αβ ) for all possible atom pairs ( Supplementary Fig. 5 ). The g αβ values, at 1,400 °C, predict that certain nearest-neighbour pairs (for example, Al-Ni, Cr-Fe and Cu-Cu) occur much more frequently than others (for example, Al-Al and Cr-Ni) and have slightly different separations ( Fig. 6e ). Similar results are seen at different temperatures [47] . These CSRO trends in the liquid can be viewed as precursors for nucleating the segregated Al-Ni-enriched, Cr-Fe-enriched and Cu-rich phases ( Fig. 2a ) [48] . The predictive nature of AIMD simulations suggests that they can be used to qualitatively guide screening single-phase HEA compositions that should minimize short-range chemical ordering or segregation in the liquid. The diffusion constants ( Supplementary Table 1 ) were obtained by plotting the mean-square displacement versus time ( Fig. 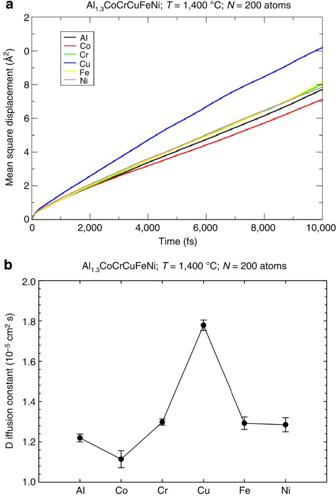Figure 7: Simulated mean-square displacements and diffusion constants. (a) Displacement plots from the present AIMD atT=1,400 °C after 30 ps. Only the data of up to 10 ps is shown in the plot for clarity. (b) Diffusion constants from the present AIMD simulations atT=1,400 °C after 30 ps. These results indicate that Cu diffuses faster than the other elements, which is consistent with the observed precipitation of Cu-rich phases (Fig. 1a–d). The error bars are based on the linear regression fitting to <R2> versus time, where five fitting analyses are performed for each temperature by varying the time of analysis. 7a ) according to the equation: Figure 7: Simulated mean-square displacements and diffusion constants. ( a ) Displacement plots from the present AIMD at T =1,400 °C after 30 ps. Only the data of up to 10 ps is shown in the plot for clarity. ( b ) Diffusion constants from the present AIMD simulations at T =1,400 °C after 30 ps. These results indicate that Cu diffuses faster than the other elements, which is consistent with the observed precipitation of Cu-rich phases ( Fig. 1a–d ). The error bars are based on the linear regression fitting to < R 2 > versus time, where five fitting analyses are performed for each temperature by varying the time of analysis. Full size image where D i is the self-diffusion constant of a species, i , and R i ( t ) and R i (0) denote the atomic positions of the species, i , at times t and t =0, respectively. The brackets denote an average over all the same species. The simulated diffusion constant for Cu is the fastest ( Fig. 7b ); it is about 60% faster than Co, which has the slowest diffusivity at T =1,400 °C, despite the fact that Cu has the highest atomic weight and similar metallic radius as Cr, Fe, Co and Ni. Similar trends in the diffusion constants was observed at T =1,600 °C (ref. 47 ). This high diffusion rate for Cu may facilitate its precipitation from the matrix, as observed in the present microscopy studies ( Figs 1 and 2 ). Combined results revealing structural evolution while cooling The present Al 1.3 CoCrCuFeNi alloy is a liquid above 1,315 °C ( Supplementary Fig. 6 ), with CSRO, revealed through both experimental PDF studies and AIMD simulations. These local structures observed in the liquid are preserved in the primary phase of the high-entropy solid solution during the initial solidification and dendritic growth [31] . It undergoes a series of microstructural changes during further cooling, progressing from a simple high-temperature structure to more complex microstructures at lower temperatures ( Table 2 ). Table 2 Evolution of structure and ordering. Full size table During the earliest stages of solidification (1,230–1,315 °C), the primary BCC phase is in equilibrium with a Cu-enriched liquid [31] , and its composition may be written as Al 1.3 CoCrCu 1-z FeNi, where z represents the Cu depletion. The upper bound of the configurational entropy, where , corresponds to z =0 and random mixing. The ‘BCC’ subscript denotes that is per mole of the BCC phase. Although the temperature dependence of z within the range of 1,230–1,315 °C was not determined, the value approaches z =0.31, based on the volume fraction of Cu-rich interdendrites observed in the room temperature microstructure. The entropy reduction, due only to the Cu depletion, is slight, such that decreases from 1.79 R to 1.78 R . A greater reduction occurs, however, due to the CSRO, which may originate from the preferred nearest-neighbour pairing in the liquid. Equation (19) was used to calculate the CSRO entropy reduction, corresponding to the case of strongly enhanced Al-TM pairs ( η Al =1, η TM =−0.28). Thus, the combination of CSRO and Cu depletion gives the lower bound, and the case of random mixing without Cu depletion gives the upper bound of the range, . In the temperature range of 1,080–1,230 °C ( Table 2 , row 3), long-range B2 ordering is detected by the presence of superstructure neutron diffraction peaks ( Fig. 5b ), in addition to the B2/BCC fundamental peaks. No other crystal phases are detected, indicating that the Cu-rich interdendrites have not yet solidified into an FCC structure. Thus, a Cu-rich liquid coexists with a Cu-depleted solid phase, identified as the high-temperature B2 phase. The solid composition is estimated as Al 1.3 CoCrCu 0.7 FeNi, such that the amount of Cu absent from the high-temperature solid is sufficient to produce the 5% interdendrite volume fraction observed in the room temperature microstructure ( Fig. 1a ). The notation B2 is used to emphasize that an average B2 structure has been determined, but the homogeneity of the phase is uncertain, and is the subject of ongoing studies. On the basis of the neutron superstructure reflections ( Fig. 5b ), the strength of the B2 long-range ordering increases as the temperature decreases, at least down to 800 °C. The lower limit is calculated using equation (3), with η Al =0.93, η TM =−0.26 (from equation 15), and the phase composition, Al 1.3 CoCrCu 0.7 FeNi. Finally, the upper limit is taken from the above CSRO calculation, giving a range of per mole of ‹B2› phase in the present temperature range of 1,080–1,230 °C ( Table 2 , row 3). In the temperature range of 600–1,080 °C ( Table 2 , row 4), the existence of the FCC diffraction peaks ( Fig. 5a ) indicates that a large fraction of the Cu has solidified, with a structure similar to that of pure Cu. Note that the melting point of pure Cu is 1,085 °C. Because the combined volume fraction of the Cu-rich interdendrites and rod-shaped precipitates is about 15% at room temperature, the present FCC diffraction peaks are attributed to the solidification of these two types of structures. In this simplified model (more detailed characterizations of the room temperature phases in the Al-Co-Cr-Cu-Fe-Ni system are found in the literature) [33] , [49] , the present B2 phase composition, in the temperature range of 600–1,080 °C, is given by Al 1.3 CoCrCu 0.1 FeNi. From equation (3), , for the ordering based on η Al =0.93 and η TM =−0.29. A spinodal structure exists below 600 °C ( Table 2 , row 5), more complex than the high-temperature structures. Using the elemental analyses obtained from X-ray EDS and APT ( Table 1 ), the spinodal B2 phase composition is Al 1.3 Co 0.79 Fe 0.51 Ni and the spinodal BCC phase composition is Co 0.21 CrFe 0.49 . The phase fractions, F BCC and F B2 , are 34 and 50%, respectively. The remaining 16% of the alloy volume is the unmixed Cu, in the form of interdendrites, rod-shaped precipitates and nanoparticles. The overall configurational entropy of mixing may be calculated as where F BCC , F B2 and F B2 represent the volume fractions of the individual phases, identified by the subscripts. As determined by comparing structural models with the diffraction trend shown in Fig. 4d , the ordering of the B2 phase (Al 1.3 Co 0.79 Fe 0.51 Ni) may be characterized by η Al =0.73, η Co = η Ni =−0.60 and η Fe =0.24. These order parameters give per mole of spinodal B2 phase, which is actually greater than the ‘disordered’ phase, where . Since the Cu-rich FCC phases give , the overall configurational entropy of mixing, per mole of the alloy, is . Table 2 summarizes all of the above microstructures, compositions, relative abundances and major features of the atomic distributions. Alloys containing several elements mixed in near-equimolar ratios, also known as high-entropy alloys, have shown exceptional engineering properties, such as high strengths at elevated temperatures [6] , [8] , [10] , ductility [16] , toughness [18] , and resistance to corrosion [20] , wear [21] and fatigue [22] . These findings have generated great interest, and intense efforts are underway to further develop high-entropy alloys for practical applications. The goal is increasingly focused on obtaining single-phase solid solution microstructures [26] , [27] , [47] , [50] . However, multiphase microstructures should not be dismissed, not only because they provide valuable test cases for understanding phase separation in high-entropy alloys, but also because many are technologically significant in their own right. For example, high-strength spinodal alloys have recently been developed using four principal elements (Al, Fe, Mn and Ni) [36] , [51] , which potentially enhances their . The success of using multiple principal elements in the development of these spinodal alloys is relevant to the high-entropy alloy research community and encouraging because it demonstrates that the strategy of using multiple principal elements is effective for developing a broad range of disordered and partially ordered alloys. Here the Al 1.3 CoCrCuFeNi material has served as a test case for studying phase separation and structural evolution, using integrated experimental and theoretical techniques. Experimental studies included high-resolution SEM, TEM and APT, revealing microstructural features across many length scales. The abundances and compositions of the individual phases were determined, using techniques such as X-ray EDS, and these results were integrated into the analyses of synchrotron X-ray and neutron scattering experiments. Ultimately, the main features of the atomic distributions, and their evolution with temperature, were experimentally determined. Theoretical AIMD studies shed further light on the atomic configurations and dynamics, showing, for example, that preferred nearest-neighbour pairing in the liquid may seed the formation of ordered B2 phases in the solid. The ordering behaviour of Al 1.3 CoCrCuFeNi was expressed in a quantitative and unambiguous fashion, instead of simply categorizing the phases according to the general structure type, such as B2. This quantitative expression is especially important in multi-element alloys, where there are several non-equivalent ways in which the elements may order to form a given structure type. In contrast to binary alloys, which may be characterized using a single-order parameter, multiple-order parameters may be required to characterize the atomic distributions. Here the complementary neutron and synchrotron X-ray scattering studies played a key role in determining these structural-order parameters, over a wide temperature range (room temperature to 1,400 °C). AIMD simulations are emerging as a predictive tool for the phase formation from the liquid [47] and have served here to identify the local-ordering trends in the liquid, particularly the CSRO, which influence the formation of the solid phases in Al 1.3 CoCrCuFeNi. Strong evidence of the local structural similarity between the liquid and solid phases has been provided by the present combined AIMD, experimental PDF and complementary temperature-dependent neutron and synchrotron X-ray diffraction studies. However, much work remains in the challenging new area of multi-element liquid alloys and their solidification behaviour. Intense research efforts are underway to develop high-entropy alloys with exceptional engineering properties. The present work addresses the fundamental need to understand the temperature-dependent elemental distributions in these multi-principal-element alloys. It was demonstrated that a set of complementary experimental and theoretical techniques could be applied to solve even the complex atomic mixing (and unmixing) behaviours of the Al 1.3 CoCrCuFeNi alloy. The observed phases, including the disordered and partially ordered solid solution structures, were quantitatively described within a unified structural model, going beyond the common practice of discretely categorizing the phases as ordered versus disordered structures. The results suggest that the high-entropy alloy-design strategy (that is, using multiple principal elements) should be considered, not only for the goal of producing single-phase solid solutions, but also for producing more complex multiphase materials with the benefit of the entropy-enhanced stability. Sample preparation Specimens were fabricated by Sophisticated Alloys (Butler, PA) using a standard arc-melting technique [8] . The composition of Al 1.3 CoCrCuFeNi (molar fraction) was selected for the present study, due to its B2-ordering tendencies. Compositional analysis was performed by Sherry Laboratories (Daleville, IN), using a direct-current plasma technique [3] , and verified that the actual composition was very close to the nominal composition. Microscopy and atom-probe tomography High-resolution SEM and TEM were performed at the Oak Ridge National Laboratory (ORNL) Center for Nanophase Materials Sciences (CNMS) [52] . The focused ion beam lamella preparation for TEM was performed using the standard liftout technique [53] . The SEM and TEM measurements were combined with the X-ray EDS to measure the elemental distribution, and EBSD to determine the crystal type and orientation of individual phases. Tomography studies were conducted at the CNMS using a local electrode atom probe (LEAP) with 37% detection efficiency. The LEAP evaporates individual atoms from a needle-shaped specimen, and computational post-processing provides a reconstruction of the atom identity (including the isotope) and location in the specimen. All samples used in the current work were derived from the same bulk ingot. Although only 37% of the evaporated atoms reach the detector and are counted, the detection sensitivity is the same for all elements, and large numbers of atoms are counted [54] . The present material, for example, has ~80 atoms within a 1-nm 3 volume and will yield about 30 counts per nm 3 . Therefore, the LEAP provides an accurate characterization of the present atomic distributions. AIMD simulations The AIMD simulations were performed at the National Energy Technology Laboratory [55] using the plane-wave pseudopotential software, Vienna Ab-Initio Simulation Package (VASP) [46] , [56] . Projector-augmented wave potentials [57] were used as supplied with VASP. The revised Perdew–Burke–Ernzerhof [58] gradient approximation to the exchange-correlation functional was used. All the calculations were carried out in a canonical ensemble, that is, a constant mole, volume and temperature, with the atomic configuration relaxation and temperature controlled by a Nose thermostat [59] . This arrangement requires the accurate determination of the densities of the liquid and solid. A cubic supercell of 200 atoms that corresponds to the Al 1.25 CoCrCuFeNi composition was built. The volume of the cell was adjusted so that the pressure is zero to reach equilibrium. The simulations were performed at the Γ point only (that is, the origin of the first Brillion zone), with a time step of 1 fs. The total simulation time is 30 ps. A ‘medium’ precision setting, as described in VASP, was used. The plane-wave cutoff energy was set at 273.2 eV. The electronic energy convergence criterion was set to 1 × 10 −4 eV per atom. The AIMD simulations were performed at temperatures of 2,000, 1,800, 1,600 and 1,400 °C in the liquid state. Previously AIMD simulations have been carried out to study the atomic structures of a variety of liquid melts [60] , [61] , [62] , [63] . Applying ordering parameters to a multi-component B2-ordered structure The B2 crystal structure may be treated as two inter-penetrating sublattices, designated by α and β [29] , [32] . In the binary B2 alloys, where the chemical formula may be written as AB, the fully ordered condition is where the A atoms reside exclusively on the α sublattice and the B atoms reside on the β sublattice. Varying degrees of ordering may be described using where η is the order parameter, x Aα is the molar fraction of the A atoms on the α sublattice, x Aβ is the molar fraction of A atoms on the β sublattice, x Bα is the molar fraction of B atoms on the α sublattice and x ββ is the molar fraction of B atoms on the β sublattice. The sublattice molar fractions ( x Aα , x Aβ , x Bα and x Aβ ) are related to the overall molar fractions, x A and x B , by and Because the molar fractions cannot be negative, η must be within the range of −1 to 1. However, the range, η =0–1, is sufficient to describe all possible ordering scenarios. Thermodynamic quantities, such as the enthalpy and configuational entropy, may be expressed in terms of x A , x B and η and calculated using the nearest-neighbour approximations [29] , [30] . Here a similar approach is used to describe multi-component alloys. Consider a B2 alloy composed of n different elements, where the overall molar fractions are given by x i , for i =1 to n . Equations (7)–(10), , ,  may be replaced by and where x i α and x i β are the molar fractions of the element, i , on the α and β sublattices, respectively, and η i is the order parameter of the element, i . Because the molar fractions, x i α and x i β , cannot be negative, all η i must be within the range of −1 to 1. Furthermore, to ensure the balanced occupation of both sublattices, the η i must satisfy Finally, the total order parameter, η , may be defined by Several different ordering scenarios are possible in the multi-component B2 phases, which may be expressed in terms of the relationships among the order parameters, η i . In the present Al 1.3 CoCrCuFeNi alloy, one scenario, which gives good agreement with the experimental data at high temperatures, has the five transition metals (Co, Cr, Cu, Fe and Ni) sharing the same ordering parameter, η TM , which is related to the Al-ordering parameter, η Al , by where x Al is the molar fraction of Al in the B2 phase. The resulting total order parameter, η , reduces to If the B2 phase has the same composition as the overall alloy, then the maximum value of η is 0.5. In general, the maximum value of η is <1, except for special compositions, such as equimolar concentrations with an even number of elements. Extending the treatment used for binary alloys [29] , thermodynamic quantities for multi-component B2 phases may be expressed using the above defined parameters, η i and x i . The molar configurational entropy of mixing is given by equation (3). Similarly, the mixing enthalpy may be calculated by summing the nearest-neighbour pairs, such that where Ω ij is the binary mixing parameter and the factor of 4 arises from the number of bonds per atom in the B2 structure [25] . The case of CSRO in multicomponent solid solutions may be treated using the pair-approximation method, which may be applied to crystal structures with two sublattices [64] . An essential feature of this method is to determine the molar fractions of first nearest-neighbour atom pairs, X i/j , for all possible combinations of the elements, i and j , on sublattices α and β, respectively. Because of the CSRO, the values of the X i/j are expected to fall between those of the randomly mixed and the long-range-ordered cases. Here the X i/j are calculated based on a mixture of random and ordered domains, where half of the atoms lie in random domains and half in the ordered domains. Similar mixtures of random and ordered domains have been observed in quenched multicomponent alloys [33] . Following the same approach as in equations (6)–(10), , , , , the X i/j may be expressed using the order parameters, η i , such that Finally, adapting the treatment of Chartrand and Pelton [64] , equation (1) may be rewritten, for the case of CSRO in a B2 structure, as Neutron scattering Neutron diffraction experiments were performed at the ORNL Spallation Neutron Source (SNS) [65] using instruments optimized for studies of local structures (NOMAD, Nanoscale-ordered Materials Diffractometer) [40] and long-range crystal ordering (POWGEN) [66] . The use of both NOMAD and POWGEN was motivated by the expectation that the present HEAs have distinct local features (for example, lattice distortions and local ordering), as well as long-range crystal order. The temperature dependence of these structures was investigated using neutron diffraction. The experiments were conducted over a wide temperature range, from room temperature to 800 °C on POWGEN and up to 1,400 °C on NOMAD, using an aerodynamic levitator ( Supplementary Fig. 4a,b ) [38] , [39] , [67] . This levitator provides a containerless environment, in which small samples (~2-mm-diameter spheres) are suspended above a conical nozzle with the flowing argon gas and heated with a 250-W CO 2 laser operating at a wavelength of 10.6 μm. For the POWGEN experiments, a conventional neutron furnace, with vanadium foil-heating elements, was used. A large sample (a 7-g polycrystalline solid) was chosen, compatible with the neutron-beam size (4 cm high and 1 cm wide). The complications of solving the multi-element B2 structure were greatly simplified, using a single parameter ( δ ) to represent the scattering contrast between the two sites in the B2 unit cell and fitting the observed data to the simplified unit cell. Here the two sites in the unit cell are characterized in terms of the average neutron scattering length where x i is the molar fraction and b i is the neutron scattering length of the i th element. In particular, the neutron scattering lengths of the two sites, α and β, are represented as and respectively. Thus, δ serves as a unitless parameter, which may be incorporated into a Rietveld refinement, and is directly related to the neutron structure factors of the B2 phase where is the structure factor of the B2 fundamental reflections, that is, those which satisfy the condition that the sum of the Miller indices ( h + k + l ) is an even number, and is the structure factor of the B2 superstructure reflections, which satisfy the condition that the sum ( h + k + l ) is an odd number. Thus, the δ parameter is equal to the ratio of the superstructure and fundamental structure factors The contrast parameter may be explicitly related to the order parameters, according to where the η i are the order parameters defined in equation (11). The observed parameter, δ obs , may be found by fitting the experimental diffraction data to a B2 crystal model, where the site occupancy is expressed in terms of δ . Thus, in accordance with equations (21) and (22), the occupancy of the site at the origin of the unit cell is given by 1+ δ and the occupancy of the site at the centre of the unit cell, (½, ½, ½), is given by 1− δ . Both sites are occupied, nominally, by the same element (here Al is chosen). This unit cell, which is clearly fictitious, reproduces the essential feature of the actual multiple principal element unit cell: a scattering contrast between the α and β lattice sites. The value of δ obs is then taken as the value of δ that gives the best fit to the experimental data. Synchrotron X-ray powder diffraction High-energy synchrotron X-ray diffraction experiments were conducted at the Argonne National Laboratory, Advanced Photon Source using beamline 6-ID-D [68] . This beamline provides monochromatic X-ray beams, using a Si (3 3 1) monochromator, in the energy range of 70–130 keV. The present powder diffraction study was conducted using 79.865 keV (0.15524 Å) X-rays, with a beam size of 1-mm 2 cross section. The Al 1.3 CoCrCuFeNi samples were ground into fine powders (<20-μm particle size) and placed in unsealed quartz capillary tubes, compatible with the high-temperature furnace provided by the beamline. The small particle size is necessary for obtaining a powder-average diffraction pattern with the small beam. Note that neutron experiments, described above, were performed with larger beam sizes, using solid, polycrystalline samples. The X-ray powder samples were heated from room temperature to 800 °C, in regular increments, to obtain the series of diffraction patterns shown in Fig. 4b . How to cite this article : Santodonato, L. J. et al. Deviation from high-entropy configurations in the atomic distributions of a multi-principal-element alloy. Nat. Commun. 6:5964 doi: 10.1038/ncomms6964 (2015).